Two principles of organization in the prefrontal cortex are cognitive hierarchy and degree of automaticity The lateral prefrontal cortex is known to be organized by cognitive hierarchies following a posterior-to-anterior gradient. Here we test whether this model applies across different cognitive domains by varying levels of cognitive hierarchy in first language, second language and non-language domains. These domains vary in their degree of automaticity with first language being the most automatic. For second language/non-language a clear gradient pattern of activation depending on the level of hierarchy is observed in the prefrontal cortex with the highest level of hierarchy recruiting its most anterior region, whereas for first language the highest level of hierarchy recruits its most posterior region. Moreover, second language/non-language and first language differ in the structural connectivity of their underlying networks. The current data strongly suggest that functional segregation of the prefrontal cortex is determined by cognitive hierarchy and the degree of automaticity. The lateral prefrontal cortex (PFC) has been segregated into subregions based on several functional characterizations [1] , [2] , [3] , [4] . Specifically, the ‘cascade model’, focusing on the temporal context, describes how executive function can be fractionated into hierarchically ordered control processes, each responsible for selecting an action based on temporal framing [5] . From this temporal dimension, one can distinguish three major cognitive control processes with increasing levels of hierarchy: contextual control (CONT) for making stimulus–response associations in the immediate context, episodic control (EPIS) for responding to stimuli depending on discrete past events, and branching control (BRAN) for selecting subsequent actions based on information conveyed by past events while intervening actions occur. The left PFC has been described as forming a cascade of subregions along the posterior-to-anterior axis based on the three levels of cognitive control: the posterior PFC (Brodmann area (BA) 44) for CONT, representing the lowest level of hierarchy; the more anterior PFC (BA 45) for EPIS, representing a mid-level of hierarchy; and the most anterior frontopolar cortex (BA 10) for BRAN, representing the highest level of hierarchy [4] , [5] , [6] . Similar to cognitive control, cross-temporal contingencies are a pivotal factor in natural language processing. The underlying mechanism of BRAN can also be applied to processing centre-embedded sentences (EMB) in language. BRAN refers to selecting an action based on pending information, which is intervened with an ongoing behavioural episode. Similarly, EMB means assigning a thematic role and keeping track of a predicate with an embedded sentence intervening. Even though the structures underlying cognitive control (BRAN) and language (EMB) are similar, they appear to recruit spatially distinct regions of the PFC: the anterior region for BRAN [6] and the posterior region for EMB [7] . Studies in the non-language (NL) domain have reported a functional gradient within the left PFC, based on the hierarchy of cognitive control and operating from the posterior region for the lowest level (CONT) to the anterior region for the highest level (BRAN) [4] , [6] , [8] , [9] . Contrastingly, in the language domain the posterior left PFC (that is, BA 44) has been observed as the ‘sensitive’ area associated with linguistic hierarchy; as the level of complexity becomes higher, activation in BA 44 increases [10] . Why this regional difference in posterior and anterior areas related to language and NL exists is an open question. Our hypothesis is that it is not the cognitive domain as such, but the degree of automaticity (that is, controlled processes versus automatic processes), which affects the regional differentiation. Most research on the cascade model was conducted using NL experiments requiring participants to associate visual symbols with new sequential rules. Usually, several training sessions were needed to familiarize participants with the tasks before the experiment. On the contrary, most studies on language hierarchy tested participants in their native language, first language (L1), which is well established and highly automated in adults. Thus, in the NL experiments, participants processed sequences that were less familiar, resulting in a controlled process drawing on general resources, whereas, in the language experiments, processing linguistic hierarchy could be accomplished by an automatic process drawing less on general resources [11] . We hypothesized that if the degree of automaticity in the hierarchical processing being tested in second language (L2) and NL domains was equal, a gradient pattern of activations along the posterior-to-anterior regions in the left PFC might be observed. To test this, Korean syllables were used as stimuli in a L2 experiment and an NL experiment involving the same German participants. Stimuli were either used as linguistic stimuli for L2 processing (after participants had learned a miniature version of Korean) or as visual symbols of colour sequence for NL processing. We used L2 rather than L1 to provide an equal degree of automaticity because L2 learning is known to engage controlled process [12] . We applied the cascade model to both domains (L2 and NL) at different hierarchical levels (that is, CONT, EPIS and BRAN). To examine the hypothesis concerning the effect of the degree of automaticity more closely, we compared the highest level of hierarchy (EMB) in L1 with the highest level of hierarchy (BRAN) in L2/NL, based on the fact that their underlying structures are identical. We hypothesized that, if the degree of automaticity is a factor in determining left PFC brain activations then different activation patterns might be observed for L1 and L2/NL, because the degree of automaticity should be relatively higher in L1 than in L2/NL. Moreover, connectivity profiles were calculated for the highest level of hierarchy in each of the three domains. We expected that a functional differentiation of the degree of automaticity between L2/NL and L1 might produce differentiation in the connectivity profiles with distinct tractograms. For the L2 experiment, participants, who had learned the miniature version of Korean, were required to judge the grammaticality of Korean sentences after completing three levels of learning (phonology, semantics and syntax). For the NL experiment, participants performed a sequence-rule judgment task after completing three levels of learning (symbol identification, colour-rule acquisition and sequence-rule application). The L2 and NL stimuli were similarly constructed with three different levels of hierarchy in the cognitive controls (CONT for the lowest level, EPIS for the middle level and BRAN for the highest level). For L1, German sentences with variable embedding (EMB structure versus nonEMB structure) and word order (object first versus subject first) were judged for grammaticality. The same German participants took part in all three experiments. Our results confirm that the cascade model of the PFC is applicable to the processing of hierarchical structure in NL sequence processing and in an early phase of L2 learning when it is still subject to controlled process, but is not applicable to native language L1 processing. Thus, there are two parallel systems dealing with a hierarchical structure; a posterior-to-anterior gradient system influenced by an increasing demand of controlled processes at the higher level of hierarchy and a posterior-only system using highly automatic syntactic processes, even at the highest level of hierarchy in the native language. This functional segregation also manifests in the structural connectivity between the ventral and the dorsal tract. Accuracy and response times The mean percentage accuracy and the total time spent learning Korean (L2) and a sequence rule (NL) are provided in Supplementary Fig. S1 . The behavioural results, mean percentage accuracy and the mean response times (RTs), from the functional magnetic resonance imaging (fMRI) studies, are provided in Supplementary Fig. S2 (for L2/NL) and Supplementary Fig. S3 (for L1). These results showed that participants performed successfully in the experiments across the three domains. Degree of automaticity index In order to measure the degree of automaticity among the processes in L1, L2 and NL, the intra-individual variability in RT, that is, the coefficient of variation in RT (CV RT ), was measured (see Supplementary Note 1 for more information). This method has been known to dissociate speed-up (improvement without increased automaticity) from restructuring (improvement with increased automaticity). According to this method, when a process becomes automatized, the CV RT is more than proportionally reduced compared with the change in RT. Therefore, if mean RT (Mean RT ) is paired with CV RT , the correlation between the two is almost zero in speed-up and significantly positive in restructuring. In the present study, CV RT showed a positive correlation with Mean RT of each condition ( r =0.72, P <0.01). EMB in L1 showed less CV RT with a shorter Mean RT compared with BRAN in L2/NL, indicating that the processing of EMB was more automatized than the processing of BRAN ( Fig. 1 ). 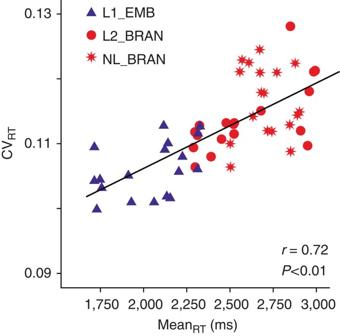Figure 1: Scatter plot showing that L1 processing is more automatic than L2/NL. Scatter plot shows the positive correlation between CVRTand MeanRT. The data from L2 and NL is clustered and mostly overlapped in the upper-right part, which means the processes in those two domains are still in the stage of controlled processing. On the other hand, the data from L1 is located in the lower-left part suggesting that our participants are highly automatized in L1 processing. All the data were obtained from the highest level of hierarchy (BRAN in L2/NL, EMB in L1) from 18 participants who participated in both L2/NL and L1 experiments (n=54). Figure 1: Scatter plot showing that L1 processing is more automatic than L2/NL. Scatter plot shows the positive correlation between CV RT and Mean RT . The data from L2 and NL is clustered and mostly overlapped in the upper-right part, which means the processes in those two domains are still in the stage of controlled processing. On the other hand, the data from L1 is located in the lower-left part suggesting that our participants are highly automatized in L1 processing. All the data were obtained from the highest level of hierarchy (BRAN in L2/NL, EMB in L1) from 18 participants who participated in both L2/NL and L1 experiments ( n =54). Full size image L2/NL experiment Brain activations elicited by the different levels of hierarchy in the cognitive controls (CONT, EPIS and BRAN) were compared across L2 and NL. We observed three dissociable subregions, moving from the posterior-to-anterior region of the left PFC as the level of hierarchy became higher ( Fig. 2 and Supplementary Table S1 ). In L2, CONT revealed activation in BA 44 (pars opercularis). The activation for EPIS in L2 was evident in the more anterior part of the PFC (BA 46) compared with CONT, and BRAN in L2 yielded the most anterior activation in BA 47 (pars orbitalis). The identical gradient-wise comparison was applied to the NL domain as well. The most posterior part of the PFC was activated in CONT in BA 6 (precentral gyrus), however, only with a more lenient threshold ( P <0.05 uncorrected voxel level). EPIS activated a more anterior region (BA 45, pars triangularis) and BRAN the most anterior region (BA 10, frontopolar cortex). Additional right hemisphere activation was observed in BA44 for BRAN in NL. Mean per cent blood-oxygen-level-dependent (BOLD) signal changes in the activated areas are plotted for each condition in Fig. 2 . 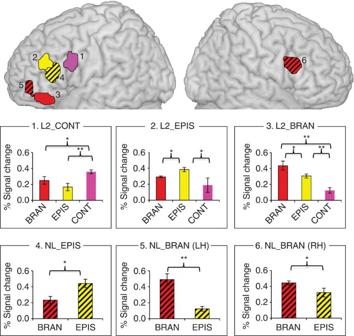Figure 2: A gradient pattern of activations depending on the levels of cognitive hierarchy across L2 and NL. Brain activations elicited by CONT, EPIS and BRAN across L2 and NL were rendered on a canonical brain provided with MRIcron software (http://www.mccauslandcenter.sc.edu/mricro/mricron/). As the level of hierarchy becomes higher (CONT, the lowest level; EPIS, the middle level; BRAN, the highest level), the activation moves from posterior-to-anterior part of the left PFC in both the L2 and NL domains. The activation of each condition was numbered with 1 for CONT, 2 for EPIS and 3 for BRAN with solid colours for L2 and with 4 for EPIS, 5 and 6 for BRAN with diagonal colours for NL. Plots of the per cent BOLD signal change in each condition within the local maxima are provided at the bottom; error bars denote s.e.m. (*P<0.05, **P<0.01,n=20, two-tailed pairedt-test. LH, left hemisphere; RH, right hemisphere). Figure 2: A gradient pattern of activations depending on the levels of cognitive hierarchy across L2 and NL. Brain activations elicited by CONT, EPIS and BRAN across L2 and NL were rendered on a canonical brain provided with MRIcron software ( http://www.mccauslandcenter.sc.edu/mricro/mricron/ ). As the level of hierarchy becomes higher (CONT, the lowest level; EPIS, the middle level; BRAN, the highest level), the activation moves from posterior-to-anterior part of the left PFC in both the L2 and NL domains. The activation of each condition was numbered with 1 for CONT, 2 for EPIS and 3 for BRAN with solid colours for L2 and with 4 for EPIS, 5 and 6 for BRAN with diagonal colours for NL. Plots of the per cent BOLD signal change in each condition within the local maxima are provided at the bottom; error bars denote s.e.m. (* P <0.05, ** P <0.01, n =20, two-tailed paired t -test. LH, left hemisphere; RH, right hemisphere). Full size image L1 experiment For a closer look at the effect of automaticity, the automatic process of L1 processing was studied and compared with the controlled process of L2/NL processing. For this, the processing of German EMB, which had the identical structure as BRAN in L2/NL, was tested in the same participant group as the L2/NL study. Additionally, the effect of word order, that is, a sentence starting with either a subject or an object, was tested in the same participants. More activation in response to the EMB than the nonEMB was observed in pars opercularis ( Fig. 3 and Supplementary Table S1 ). This result showed that, in contrast to L2/NL, the activation obtained from the highly automatic process (L1) was located in the posterior region of the PFC. The activations related to the processing of word order were shown in precentral and inferior frontal gyrus (IFG) ( Supplementary Fig. S4 ). 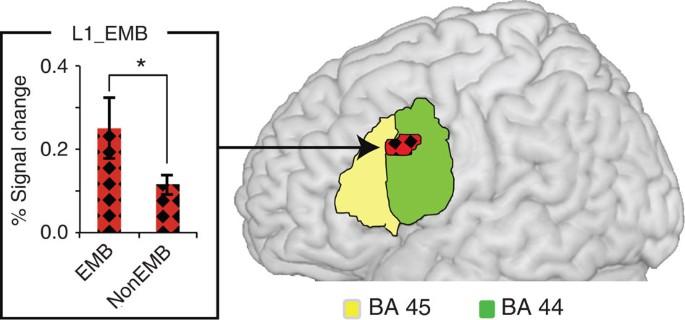Figure 3: The activation in the posterior region for the automatic processing. The activation elicited by main effect of EMBEDDING in L1 is overlaid on the cytoarchitectonic map of BA 44 (green) and BA 45 (yellow). Plot of the per cent BOLD signal change from activated clusters in each condition is provided in the bar graphs on the left; errors bars denote s.e.m. (*P<0.01,n=18, two-tailed pairedt-test) EMB, centre-embedded sentences; NonEMB, non-embedded sentences. Figure 3: The activation in the posterior region for the automatic processing. The activation elicited by main effect of EMBEDDING in L1 is overlaid on the cytoarchitectonic map of BA 44 (green) and BA 45 (yellow). Plot of the per cent BOLD signal change from activated clusters in each condition is provided in the bar graphs on the left; errors bars denote s.e.m. (* P <0.01, n =18, two-tailed paired t -test) EMB, centre-embedded sentences; NonEMB, non-embedded sentences. Full size image Singular value decomposition We extracted the each individual’s xyz-coordinates from the Montreal Neurological Institute (MNI) space of the peak activations in CONT, EPIS, BRAN in L2/NL and transformed them into an optimal coordinate system using singular value decomposition (see Supplementary Note 2 for more information). A factorial analysis of variance on the coordinates of the activation peaks between DOMAINS (L2 and NL) and HIERARCHY (CONT, EPIS, BRAN) showed a main effect of HIERARCHY ( F 2,100 =2313.2, P <0.001). No significant main effect was found for the factor DOMAIN ( F 1,100 =0.028, P =0.868). No significant interaction effect was observed between DOMAIN and HIERARCHY ( F 1,100 =5.96, P =0.16). The post hoc test was conducted on variables of hierarchical levels. The Bonferroni tests showed that the comparison between the two conditions (CONT versus EPIS, EPIS versus BRAN, BRAN versus CONT) showed significant differences in terms of their peak activation areas ( P <0.001 in all the comparisons). Correlation between automaticity and activation To ensure that the degree of automaticity elicited a regional difference between posterior and anterior activations within the left PFC, we conducted a correlation analysis between individual CV RT and the per cent BOLD signal change from the peak activation areas in a controlled process (BA 47 in L2 and BA 10 for NL) and an automatic process (BA 44 for L1) ( Fig. 4 ). BA 10 and BA 47 showed higher BOLD signals with the increase of CV RT , which means that these areas showed more activations when they were involved with the process inherent to the low degree of automaticity (high CV RT ). On the contrary, the BOLD signals from BA 44 was negatively correlated with CV RT indicating that this area was more activated when it was related to the highly automatic process (low CV RT ). 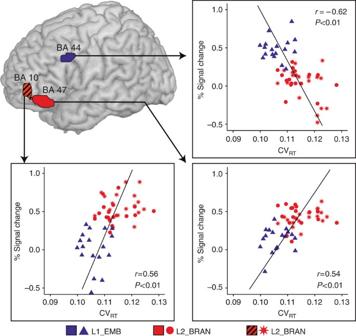Figure 4: Influence of the degree of automaticity on the activation areas of the left PFC. Activations for the highest level of hierarchy in L2 (BA 47), NL (BA 10) and L1 (BA 44) were rendered on a canonical brain provided with MRIcron software (http://www.mccauslandcenter.sc.edu/mricro/mricron/) on the top left. All the peak activations were provided with a scatter plot of each individual’s CVRTas a function of the per cent BOLD signal changes from the regions (n=54). L1_EMB, center embedded sentences in the first language; L2_BRAN, branching control in the second language; NL_BRAN, branching control in the non-language. Figure 4: Influence of the degree of automaticity on the activation areas of the left PFC. Activations for the highest level of hierarchy in L2 (BA 47), NL (BA 10) and L1 (BA 44) were rendered on a canonical brain provided with MRIcron software ( http://www.mccauslandcenter.sc.edu/mricro/mricron/ ) on the top left. All the peak activations were provided with a scatter plot of each individual’s CV RT as a function of the per cent BOLD signal changes from the regions ( n =54). L1_EMB, center embedded sentences in the first language; L2_BRAN, branching control in the second language; NL_BRAN, branching control in the non-language. Full size image Structural imaging results The functional segregation between the automatic and controlled processes within the left PFC was also investigated in terms of the structural connectivity. The peak coordinates of individual activations in the highest level of hierarchy, that is, BRAN for L2/NL and EMB for L1, were taken as the seed points for the tractograms. A clear dissociation was demonstrated between L2/NL and L1 regarding a structural connectivity; BA 47 (L2) and BA 10 (NL) connects with the temporal lobe via the extreme capsule fibre system (ECFS) and BA 44 (L1) connects with the superior temporal region via the arcuate fasciculus (AF) and with IFG via short-range association fibres ( Fig. 5 ). These data revealed that the processing difference depending on the level of automaticity was manifested in the structural connectivity between the ventral and the dorsal tract. 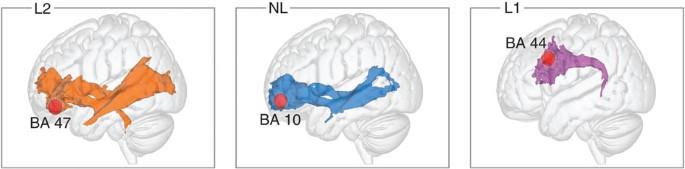Figure 5: Differential tractograms for the peak activations from different domains. The peak activations from the highest level of hierarchy (BRAN for L2/NL, EMB for L1) were taken as the seed points for the tractogram. Red circles denote the activation peaks in each condition. Orange: tractograms from BA 47 in the second language; blue: tractograms from BA 10 in the non-language; purple: tractograms from BA 44 in the first language. Figure 5: Differential tractograms for the peak activations from different domains. The peak activations from the highest level of hierarchy (BRAN for L2/NL, EMB for L1) were taken as the seed points for the tractogram. Red circles denote the activation peaks in each condition. Orange: tractograms from BA 47 in the second language; blue: tractograms from BA 10 in the non-language; purple: tractograms from BA 44 in the first language. Full size image We investigated the organization of the left PFC across different cognitive domains (L1, L2 and NL) with respect to its hierarchical structure and the degree of automaticity. We hypothesized that the left PFC is hierarchically structured in a similar way across the language and NL domains, but only if the degree of automaticity of processing is equal (L2 and NL) and not when processes are highly automatic (L1). This hypothesis was confirmed by the following findings. First, in an experiment where three different levels of cognitive control (CONT, EPIS and BRAN) were implemented in a rule-learning task in two different domains (L2 and NL), keeping the degree of automaticity at a similar level, we found that both L2 and NL activated the left PFC in a hierarchical manner; moving from posterior-to-anterior regions as the level of hierarchy increases ( Fig. 2 ). Second, to investigate the effect of the degree of automaticity more closely, we compared L1 (representing an automatic process) with L2/NL (representing controlled processes) at the highest level of hierarchy. In contrast to L2/NL, the automatic L1 process did not map onto the gradient pattern because the highest level of hierarchy in L1 activated the most posterior portion of the left PFC, the pars opercularis ( Fig. 3 ). Third, to verify that the degree of automaticity elicited a regional difference between posterior and anterior activation within the left PFC, we conducted a correlation analysis between individual CV RT and the per cent BOLD signal change from the activated foci of L2/NL (BA 47/BA 10) and L1 (BA 44). Although a positive correlation was observed in BA 10 and BA 47 from BRAN, a negative correlation was found in BA 44 from EMB; strongly suggesting that the regional difference in anterior and posterior areas was determined by the degree of automaticity ( Fig. 4 ). Fourth, this regional difference was also reflected in structural connectivity patterns to the temporal cortex: we observed the ventral pathway (ECFS) for L2/NL and the dorsal pathway (AF) for L1 ( Fig. 5 ). To the best of our knowledge, the present study is the first attempt to approach the structure of the left PFC from these two different principles, namely, cognitive hierarchy and degree of automaticity. As expected from the cascade model, the functional fractionation from posterior-to-anterior regions of the left PFC was clearly observed in the different levels of hierarchies in NL. The most anterior part of the PFC (BA 10), which is known to be a BRAN specific area [13] , was selectively activated in BRAN. BA 10 has been consistently shown to activate when implicated in tasks where participants have to suspend information processing temporarily while performing a secondary task in prospective memory [14] or monitoring [15] . The peak coordinates of EPIS in our study (−41, 27, 19)—which are converted into Talairach coordinates—are located adjacent to those of Koechlin’s cascade model (−40, 32, 20) [6] . Here, we observed a specific activation of CONT only with a lower threshold in BA 6 (precentral gyrus) in NL. This may be due to the relatively low level of cognitive control in CONT compared with the other conditions. In the cascade model, BA 6 is known to be related to sensorimotor control, which integrates signals from stimuli to decide how to act at the lowest level of hierarchy [4] , [5] . In our study, even though participants were required to associate the stimulus with its context in CONT, the processing demand for the task may have been similar to simple sensorimotor control, resulting in the activation in BA 6. Intriguingly, additional activation was observed in the IFG of the right hemisphere for BRAN in NL. Previous studies elucidating the neural correlates of rule learning in the NL domain, that is, visuospatial symbols, nongrammatical sequences and finite state grammar of consonant strings, obtained a significant activation in the right IFG [16] . Some studies on sign language have also found enhanced activation in this area [17] . Putting these results together, the right IFG seems to be involved in abstracting structural knowledge from the visuospatial domain; it was already known that the right hemisphere is specialized for processing visuospatial information [18] . Considering that our NL learning pertains to extracting sequential rules by processing visuospatial information, the present result fits in well with previous studies. Here, we successfully applied the three levels of cognitive control from the cascade model to the language domain and the NL domain for the first time. To what extent the participants of our study were truly involved in L2 learning may be a matter of discussion. However, based on the theories about the optimal linguistic environment for adult L2 learners, all the learning procedures in our study were conducted in a formal environment where language input could be controlled depending on learners’ performance with an interaction [19] , [20] . We, therefore, stand by the assertion that our experimental settings for L2 meet all the requirements for L2 learning (see Supplementary Note 3 ). Thus, the present results are taken to suggest that the cascade model can be applied to not only executive control in action selection, but also the processing of hierarchical sequences in L2 in a similar way. The processing of structural hierarchy in L2 yielded a clear distinction in the activated areas in CONT, EPIS and BRAN. The posterior region (BA 44) and the middle region (BA 46) have been already specified for the effects of CONT and EPIS in other studies with successively presented visual stimuli [4] , [6] . The most anterior region (BA 47) in BRAN has been shown to manifest as a crucial area for hierarchical processing in cognitive domains where processes are less automatic, such as mathematical formulae [21] . Therefore, the brain region involved in more cognitive, demanding tasks in L2 maps onto the posterior-to-anterior gradient in the PFC. We compared L2/NL with L1 based on the hypothesis that the degree of automaticity might influence activation patterns across the domains. At this point, it might be worth considering the degree of automaticity in some detail. A large number of studies have generalized the effects of practice on skilled behaviour: it leads to faster and more stable latencies in performance [22] , [23] , [24] . With respect to this, CV RT has been specifically used to investigate the development of automaticity in L2 acquisition in various tasks, for example, vocabulary acquisition [25] , lexical decision [26] , semantic priming [23] and attention control [27] . In our study, we obtained a strong positive correlation between Mean RT and CV RT ; EMB in L1 showed less variability and shorter RTs than BRAN in L2/NL ( Fig. 1 ), suggesting that the process was more automated in L1 than in L2/NL. The degree of automaticity and its relation to anterior/posterior activations in the left PFC have been investigated in a number of previous studies. It has been observed that L2 learners must compensate for their lower efficiency by deploying additional cognitive resources, such as working memory, attention and monitoring. Thus, they recruit neural structures related to more general cognitive controls in addition to those for language-specific process [28] . For example, L2 learners showed activations in not only the L1-related prefrontal networks but also in more anterior areas, such as BA 9, 46, 47 (refs 29 , 30 ) and the same holds for L1 processing in childhood when processes are not yet fully automatic and proficient [31] . On the other hand, it has been reported that the activity in the anterior PFC decreased for high proficiency L2 learners, suggesting that the reduced activation in this area may be linked to the decrease of processing demands inherent to the task [32] . All these studies fittingly explain our results regarding the divergence of peak activation between L2/NL and L1. More specifically, the correlation between the individual CV RT and the per cent BOLD signal change in the peak areas of BRAN in L2/NL and EMB in L1 adds additional support to the idea that the degree of automaticity is related to the regional difference within the left PFC. The positive correlation observed in the anterior region of the PFC highlights the nature of L2/NL processing, namely, a controlled process with low proficiency. Furthermore, the equal degree of task demands between L2 and NL is reflected in similarly clustered data ( Fig. 4 ). In line with this, the negative correlation found in the posterior region explains that the activation confined to the posterior PFC is related to a highly automatized processing with high proficiency in L1. The activation of BA 47 in BRAN in L2 deserves some discussion in terms of its functional role. A large body of studies of L1 using English as a test language found enhanced activity in Broca’s area (that is, left BA 44 and BA 45 extending to BA 47), suggesting that this area is activated by syntactic manipulations and task demands [33] . However, it has been also postulated that BA 47, usually combined with BA 45, supports the retrieval of semantic information and the processing of semantic relationships between words in sentences [34] , [35] . This area has also been observed to activate more when there is an increasing demand for the top–down retrieval of semantic association in languages whose syntactic demands are low, such as Chinese [36] . If we look at the task of L2 learning more closely, it appears that the processing of BRAN is partially dependent on the semantic association between a subject and its following verb form; for example, connections between a subject and prefinal endings for subject honorification, temporal adverb or verb tense. Thus, even after (or while) building a sentence structure, participants may have been involved in the processing of semantic aspects, which yielded the activation in BA 47. It has been known that BA 47/45 is connected to the temporal lobe via the ECFS, as a ventral pathway, supporting the processing of semantic information [37] and syntactically simple sentences [33] . As mentioned above, the task of BRAN in L2 may be related to processing semantic information, as well as building up a sentence structure. Here, semantic information could be transferred from BA 47, via the ventral pathway and through the ECFS, to the temporal cortex. Interestingly, a ventral pathway starting out from BA 10 was observed in NL. A feasible explanation for the involvement of this pathway may be that participants have developed strategies by associating symbols with information previously stored in long-term memory for efficient learning requiring top–down processes. The dorsal pathway from BA 44 to the superior temporal region via the AF is known to be involved in hierarchical structure processing (that is, syntactic processing) especially when the sentences are complex [37] . This argument is compatible with our results, because participants had to process a phrase structure grammar in the form of EMB, which usually demands more cognitive resources than finite state grammar [34] . From the current data we conclude that two principles of organization underlie the fractionation of the network of brain regions in the PFC: cognitive hierarchy and degree of automaticity. L2 and NL experiment Twenty participants (10 males, 10 females; 19–29 years, 23.4±2.4 years) with no history of neurological or psychiatric disease gave written, informed consent to participate in the L2 and NL study. They were all right-handed (mean LQ=97.2, s.d.=7.8) [38] and native speakers of German. No participants had experience of learning Korean or any other Asian language. The study was approved by the Research Ethics Committees of the University of Leipzig. The learning procedure applied to both L2 and NL is explained in more detail in Supplementary Methods . For L2 learning, participants learned a miniature version of Korean that was modified to contain invented vocabulary with easy pronunciation and simple grammar. This modified version of Korean guaranteed successful behavioural performance after a short period of training [39] . Learning comprised three different levels covering syllable, vocabulary and grammar learning (see Supplementary Table S2 for syllable learning, Supplementary Table S3 for vocabulary learning, Supplementary Table S3 and Fig. 6a for grammar learning). For NL learning, new symbols (Nero and Fero) were devised, which were borrowed from Korean vowels and consonants, respectively. NL learning comprised three levels: symbol (Nero/Fero) identification, Nero colour-rule acquisition and Fero sequence-rule application (see Supplementary Table S4 for symbol identification, Supplementary Table S5 for Nero colour-rule acquisition Supplementary Table S6 and Fig. 6b for Fero sequence-rule application). 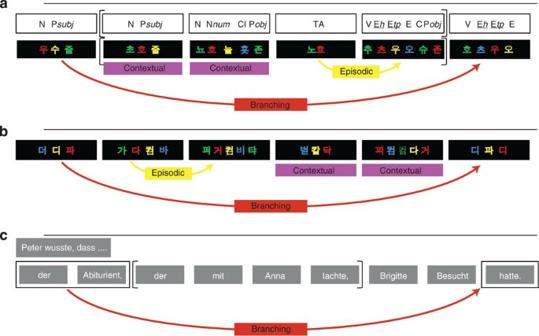Figure 6: Schematic of the three cognitive controls in different domains. (a) A miniature Korean sentence is depicted (with grammatical explanations above it). The bracketed part indicates an embedded structure. The underlined Ehor Etpcan be omitted depending on the subject or tense of a sentence. For BRAN, the first subject (: father) should coincide with the last verb in terms of honorification. The temporal adverb (: yesterday) influences the choice of verb tense for the next verb phrase in EPIS. For CONT, ordering ((N+Psubj), (N+Nnum+Cl)), or the type of classifier (: Cl for flower), are contained and processed within the phrase itself without having to refer to other phrases. Translation: ‘Father liked that mother bought one flower yesterday.’ (b) Fero sequence rule. In the case of BRAN, the first Fero symbol of the first chunk () belongs to F2, so that the Nero colour rule of the first chunk also applies to a subsequent chunk starting with F2 (6th chunk). In EPIS, the second chunk starts with F1 () and thus its Nero colour sequence is also applicable to the next chunk. In CONT, the fourth and the fifth chunks begin with F3 (), so that the Nero colour rule of the chunks is applied to only the current ones. (c) A German-embedded sentence has the same structure as in BRAN. Translation: ‘Peter knew that a high school graduate who laughed with Anna had visited Brigitte.’ Figure 6: Schematic of the three cognitive controls in different domains. ( a ) A miniature Korean sentence is depicted (with grammatical explanations above it). The bracketed part indicates an embedded structure. The underlined E h or E tp can be omitted depending on the subject or tense of a sentence. For BRAN, the first subject ( : father) should coincide with the last verb in terms of honorification. The temporal adverb ( : yesterday) influences the choice of verb tense for the next verb phrase in EPIS. For CONT, ordering ((N+P subj ), (N+N num +Cl)), or the type of classifier ( : Cl for flower), are contained and processed within the phrase itself without having to refer to other phrases. Translation: ‘Father liked that mother bought one flower yesterday.’ ( b ) Fero sequence rule. In the case of BRAN, the first Fero symbol of the first chunk ( ) belongs to F2, so that the Nero colour rule of the first chunk also applies to a subsequent chunk starting with F2 (6th chunk). In EPIS, the second chunk starts with F1 ( ) and thus its Nero colour sequence is also applicable to the next chunk. In CONT, the fourth and the fifth chunks begin with F3 ( ), so that the Nero colour rule of the chunks is applied to only the current ones. ( c ) A German-embedded sentence has the same structure as in BRAN. Translation: ‘Peter knew that a high school graduate who laughed with Anna had visited Brigitte.’ Full size image Participants were given 30 min training before the actual scanning session to brush-up on what they had learned for 2 days previously. Across the domains, experiments consisted of two sessions and each session comprised 52 sentences in L2 or 52 sequences in NL. Sentences/sequences were composed of six phrases/chunks having two CONT, one EPIS and one BRAN. More explanations about the L2/NL conditions are provided in Supplementary Methods . Sentences/sequences started with a baseline condition (BASE) in which several Xs (a minimum of two and a maximum of six) were shown and participants were required to simply push the response button. By having BASE, the effect of visual processing and motor responding could be subtracted out for fMRI analysis. Six phrases/chunks in a sentence/sequence were visually presented one by one and each stimulus was shown for 3 s, jittered by 0, 0.5, 1, 1.5 or 2 s. The three conditions were randomly positioned in the sentences/sequences. Participants were asked to judge whether a phrase or a chunk was correct or incorrect via button press. Twenty percentage of the total sentences/sequences had no errors or errors in two or three conditions. Mean sentence/sequence asynchrony was 28 s and one session lasted for 1456, s, resulting in ~50 min for two sessions. Stimuli were projected through an LCD projector onto the back of a screen. Participants viewed the images on the screen above their heads through a mirror attached to the head-coil. Analysis and visualization were performed using SPM8 software ( http://www.fil.ion.ucl.ac.uk/spm/ ). The procedure of preprocessing is explained in Supplementary Methods . We performed first- and second-level statistics using the general linear model. In the first-level analysis, each participant’s hemodynamic responses were modelled with a box-car function. Six motion parameters (realignment parameters: translation along, and rotation around, the x y and z axes) were added as regressors. Overall patterns of activations were first obtained by a fixed-effect analysis on data pooled over all participants. Statistical inferences on task and condition differences were then performed with a random effect model to render the results of the inference generalizable to the population. Condition-specific effects involved creating contrast images of each condition (CONT, EPIS and BRAN) compared with BASE for each subject. These contrast images were then entered into a second-level random effect analysis. Based on the hypothesis, we tried to observe activations that increased gradually as the level of hierarchy became higher in L2 and NL, separately. Therefore, contrasts of each level were defined as (EPIS>CONT) for EPIS, (BRAN>(EPIS CONT)) for BRAN. For CONT, CONT>BASE was used. Unless mentioned otherwise, contrasts were initially thresholded at P <0.001 uncorrected and only activations that survived P <0.05 FWE (family wise error) at cluster level involving at least 25 significant voxels were reported. Average per cent BOLD signal changes in the contrast images of the three main conditions (CONT, EPIS and BRAN) in L2 and NL were calculated using Marsbar ( http://marsbar.sourceforge.net/ ). Additionally, to examine the anterior–posterior regional differences with respect to the degree of automaticity, a Pearson’s correlation coefficient was calculated between all the participants’ CV RT and their BOLD signal changes in the peak activations of BRAN in L2/NL and EMB in L1. L1 experiment Among the 20 participants who already took part in the L2/NL experiments, 18 participants (8 males, 10 females; 19–29 years, 22.7±4.2 years) also participated in the L1 study. Written informed consent was obtained from all participants. The study was approved by the Research Ethics Committees of the University of Leipzig. fMRI scanning for the L1 experiment was performed three months after the first study (L2 and NL). The experiment had a 2 × 2 design for a language experiment investigating the processing of syntactic hierarchy with factors WORD ORDER (subject first [S] versus object first [O]) and EMBEDDING (EMB versus non-embedded sentences [NonEMB]), resulting in four experimental conditions of EMB-S, EMB-O, NonEMB-S and NonEMB-O. More explanation for L1 condition was provided in Fig. 6c and Supplementary Methods . A sentence started with a lead-in phrase, ‘Peter wusste, dass (Peter knew that)’, shown for 0.5 s and this was followed by 9 words, that is, 10 words in total, presented one by one across all conditions. The lead-in phrase was jittered between 0 and 800 ms. The duration for each word was 0.5 s with an inter-stimulus interval of 0.1 s. After the last word disappeared, either a blank screen was shown until the next sentence appeared or a probe sentence stayed for 3.6 s in 20% of sentences from each condition to confirm that participants fully understood the sentences and remained alert. Participants were required to judge whether the meaning of the probe sentence was identical with the sentence and answered with yes/no via button press. Mean sentence onset asynchrony was 11.2 s. Two fMRI-scanning sessions were administered and one session consisted of 23 sentences for each sentence condition and 23 null events (a blank screen presented for 11.2 s), in total there were 115 trials for one session. Total scanning time was ~43 min. The order of sessions, conditions and null events were randomized. Semantic information carried by the sentences was equated across EMB-S and EMB-O as well as NonEMB-S and NonEMB-O by using the same vocabularies. Preprocessing was performed in the same way as in the L2/NL experiment, except for 808 volumes per one scanning session. We performed first- and second-level statistics using the general linear model. In the first-level analysis, each participant’s hemodynamic responses were modelled with a box-car function with 5.9 s duration for sentences-only trials and 9.6 s duration for the sentences with probe trials. Six motion parameters were added as regressors. For the second-level analysis, the statistical inferences for the brain activations of the main effects and interactions were confined to the volume of interest in the posterior left IFG (BA 44 and BA 45) (see Supplementary Methods for more details about volume of interest). Average per cent BOLD signal changes were calculated using Marsbar ( http://marsbar.sourceforge.net/ ). The contrast images of the four main conditions (EMB-S, EMB-O, NonEMB-S and NonEMB-O) in each participant were used for a within-subject analysis of variance with two factors EMBEDDING and WORD ORDER. A main effect of EMBEDDING and WORD ORDER was identified with the contrast of ((EMB-O+EMB-S)>(NonEMB-O+NonEMB-S)] and [(EMB-O+NonEMB-O)>(EMB-S+NonEMB-S)), respectively. Contrasts were identically thresholded with L2/NL experiment. Details regarding behavioural data analysis, fMRI and diffusion MRI (dMRI) data acquisition, dMRI data analysis (white matter tractography) for L1, L2 and NL can be found in the Supplementary Methods . How to cite this article: Jeon, H.-A. et al. Two principles of organization in the prefrontal cortex are cognitive hierarchy and degree of automaticity. Nat. Commun. 4:2041 doi: 10.1038/ncomms3041 (2013).